Single-molecule identification via electric current noise Label-free and real-time single-molecule detection may aid the development of high-throughput biosensing platforms. Molecular fluctuations are a source of noise that often hinders single-molecule identification by obscuring the fine details of molecular identity. In this study, we report molecular identification through direct observation of quantum-fluctuation-induced inelastic noise in single organic molecules. We investigated current fluctuations flowing through a single molecule that is chemically connected to two electrodes. We found increased current oscillations synchronous to electric field excitations of characteristic molecular vibrational modes that contribute to inelastic electron tunnelling. This finding demonstrates a large contribution of charge interaction with nuclear dynamics on noise properties of single-molecule bridges and suggests a potential use of inelastic noise as a valuable molecular signature for single-molecule identification. Recent advances in single-molecule detection techniques have revolutionized our understanding of biological phenomena and opened new opportunities for human gene analysis [1] , [2] , [3] , [4] , [5] , [6] . Unlike ensemble average measurements of macroscopic properties, molecular fluctuations generate a noise that often becomes a serious impediment for identifying important single-molecule signatures. In stark contrast, human sensory apparatus deals with the stochastic nature of biological systems by leveraging the unique ability to use noise for detecting weak electrical signals (via the stochastic resonance mechanism) [7] , [8] . Likewise, noise analyses have provided valuable insights into single-molecule science. In particular, shot noise measurements have proven to be a powerful method for evaluating the Fano factors, as well as the number and transparency of channels for charge transmission in individual molecules [9] , [10] . In spite of these sophisticated experiments, little is known about noise characteristics in the inelastic regime, in which conducting electrons interact with molecular vibrational degrees of freedom. Here, we report the observation of inelastic contributions to current noise in single organic molecules connected to two metal electrodes. We analysed conductance fluctuations in a current-carrying molecular bridge under a high field. We found stepwise increases in the current oscillation amplitudes at distinct voltages. Our results suggest that this field-induced current noise originates from inelastic excitations of characteristic vibration modes inherent to target molecules, and thus manifests itself as a valuable molecular signature for single-molecule identification. Current versus bias voltage in single-molecule junctions We explored high-field conductance fluctuations in 1,6-hexanedithiol (HDT) single molecules trapped between two Au nanoelectrodes (HDT single-molecule junctions) using a self-breaking technique at 4 K under a low applied voltage of 0.2 V ( Fig. 1a,b ; Supplementary Figs S1–S3 ). 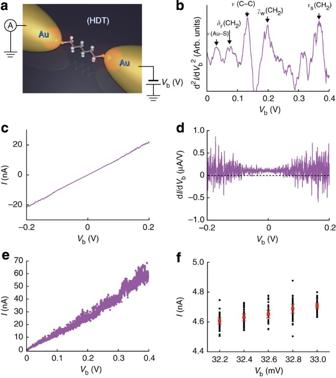Figure 1: A measurement scheme for characterizing current fluctuations in single-molecule junctions. (a) A schematic illustration showing a measurement circuit used to investigate the high-field conductance fluctuations in Au–HDT–Au single-molecule junctions at 4.2 K. (b) IET spectrum of the HDT single-molecule junction formed by a self-breaking technique at 4.2 K. The peaks indicated by arrows can all be assigned to the IETS-active molecular vibrational modes (Supplementary Figs S1–S3for details). (c) An example ofI–Vbcharacteristics acquired for HDT single-molecule junctions at 1.3 mG0conductance state. (d) Differential conductance numerically derived from theI–Vbcurve inb, revealing considerable fluctuations at highVbregimes. (e) 50-point current measurements conducted for evaluating the bias voltage-induced conductance fluctuations observed in HDT single-molecule junctions. (f) A magnified view of the plots ine. Black and red dots are the 50-point current data measured at eachVband the corresponding average current <I>. Error bars denote s.d. Figure 1c shows an I – V b curve measured by a direct current (DC) method. The linear characteristics represent tunnelling electron transport through an HDT molecule, with a large highest occupied molecular orbital-lowest unoccupied molecular orbital (HOMO-LUMO) gap exceeding 6 eV that yields a high carrier injection barrier at the metal–molecule interfaces when bonded to Au electrodes. In addition, we observe that current tends to become unstable with increasing V b . Correspondingly, the numerical differential conductance exhibits considerable fluctuations at high- V b regimes ( Fig. 1d ). We note that the magnitude of the fluctuations is enhanced with increasing V b . Figure 1: A measurement scheme for characterizing current fluctuations in single-molecule junctions. ( a ) A schematic illustration showing a measurement circuit used to investigate the high-field conductance fluctuations in Au–HDT–Au single-molecule junctions at 4.2 K. ( b ) IET spectrum of the HDT single-molecule junction formed by a self-breaking technique at 4.2 K. The peaks indicated by arrows can all be assigned to the IETS-active molecular vibrational modes ( Supplementary Figs S1–S3 for details). ( c ) An example of I – V b characteristics acquired for HDT single-molecule junctions at 1.3 m G 0 conductance state. ( d ) Differential conductance numerically derived from the I – V b curve in b , revealing considerable fluctuations at high V b regimes. ( e ) 50-point current measurements conducted for evaluating the bias voltage-induced conductance fluctuations observed in HDT single-molecule junctions. ( f ) A magnified view of the plots in e . Black and red dots are the 50-point current data measured at each V b and the corresponding average current < I >. Error bars denote s.d. Full size image Electric field dependence of current noise in HDT To elucidate the underlying mechanism responsible for the electric-field-induced conductance fluctuations in single HDT molecules, we carried out consecutive 50 current measurements per V b condition at a sampling rate of 30 Hz during a bias sweep in a range of −0.38 V≤ V b ≤0.38 V ( Fig. 1e ) and examined their average current < I > and current noise σ ( Fig. 1f ). 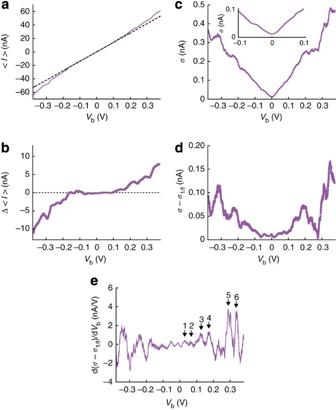Figure 2: Charge transmission and current fluctuations in a single-molecule tunnelling junction. (a) <I>–Vbcharacteristics obtained for an HDT single-molecule junction at 4 K. The dotted lines are the elastic current assumed to increase linearly withVb. (b) Δ<I> plots derived from <I>–Vbcurve ina. (c) σ versusVbplots acquired for an HDT single-molecule junction at 4.2 K. (d) σ plots after subtracting 1/f-like contributions σ1/f. (e) The d(σ–σ1/f)/dVb–Vbcurve obtained numerically fromd. The characteristic peaks are labelled numerically. < I > is plotted as a function of V b in Figure 2a . We obtained linear < I >– V b characteristics analogous to the I – V b curve shown in Figure 1c . Subtracting the elastic tunnelling current I e from < I > yields the inelastic component Δ< I >=< I >– I e [11] , [12] . We estimated I e from a linear fit to the < I >– V b curve in a low bias range of −0.005 V≤ V b ≤0.005 V; nonlinearity of elastic tunnelling contributions is anticipated to be negligibly small because of the relatively high tunnelling barrier at the electrode–molecule links expected for the insulating molecular wire of HDTs ( Supplementary Fig. S4 ). By extrapolating linear I e – V b to high biases (dotted line in Fig. 2a ), we extracted Δ< I > and plotted with respect to V b ( Fig. 2b ). The fact that |Δ< I >| rises above 0 A with increasing V b implies opening of active inelastic channels, rendering an increase in transmission of HDT molecules [11] , [12] , [13] . Figure 2: Charge transmission and current fluctuations in a single-molecule tunnelling junction. ( a ) < I >– V b characteristics obtained for an HDT single-molecule junction at 4 K. The dotted lines are the elastic current assumed to increase linearly with V b . ( b ) Δ< I > plots derived from < I >– V b curve in a . ( c ) σ versus V b plots acquired for an HDT single-molecule junction at 4.2 K. ( d ) σ plots after subtracting 1/ f -like contributions σ 1/ f . ( e ) The d(σ–σ 1/ f )/d V b – V b curve obtained numerically from d . The characteristic peaks are labelled numerically. Full size image Meanwhile, σ is found to increase with V b , manifesting more pronounced current fluctuations in the HDT single molecule under high field ( Fig. 2c ). Moreover, although somewhat obscure at a low- V b region, σ– V b plots demonstrate a staircase-like voltage dependence. We first note an overall linear response of σ with respect to V b . This feature is generally interpreted by Hooge's empirical rule established for bulk materials that states a linear response of the resistance fluctuation-induced 1/ f noise amplitude to current [14] , [15] . The validity of this rule in atomic- and molecular-scale conductors has been examined recently for various nanomaterials, such as carbon nanotubes, graphenes and atom-sized contacts [16] , [17] , [18] , [19] . We subtracted the 1/ f -like noise σ 1/ f by linear fitting to σ– V b plots in the positive and negative V b regimes. The resulting (σ−σ 1/ f )– V b plots reveal clear steps at distinct V b ( Fig. 2d ). Measurements on another 40 HDT single-molecule bridges yielded similar results. Numerical differentiation as shown in Figure 2d yields a spectrum with pronounced peaks that emerged at positions corresponding to the σ steps ( Fig. 2e ). These peaks are located at V p =30, 66, 127, 172, 300 and 337 mV in the positive side and at V p =−31, −79, −127, −199, −298 and −369 mV in the negative side ( Table 1 ). The spectrum is therefore almost symmetric with bias polarity. Table 1 Peaks in the σ-spectrum for an Au–HDT–Au single-molecule junction and an Au–Au single-atom chain. Full size table We examined the reproducibility of the characteristic σ steps by statistically analysing σ– V b characteristics for 41 HDT single-molecule bridges at 1.3 m G 0 . A histogram constructed with V p data extracted from the σ spectrum of single HDT molecules contains several peaks at almost symmetric positions with respect to zero bias ( Fig. 3 ). As we see in Table 2 , the statistical V p distribution fairly reproduces the σ spectrum shown in Figure 2e . 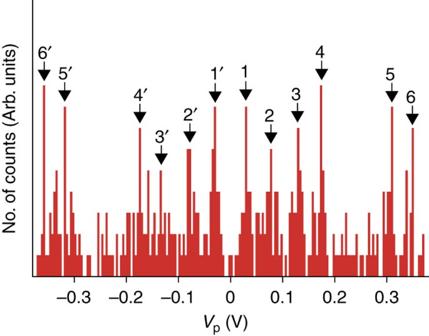Figure 3: A peak voltage histogram constructed withVpdata extracted from the σ spectra of 41 HDT single-molecule junctions formed at 4.2 K. Peaks are numbered as 1–6 and 1′–6′ in the positive and the negative side, respectively. Figure 3: A peak voltage histogram constructed with V p data extracted from the σ spectra of 41 HDT single-molecule junctions formed at 4.2 K. Peaks are numbered as 1–6 and 1′–6′ in the positive and the negative side, respectively. Full size image Table 2 Peaks in the V p histogram of Au–HDT–Au single-molecule junctions. Full size table Noise characteristics of gold single-atom contacts It is interesting to note that the σ peak profile agrees with what appears in the inelastic electron tunnelling (IET) spectrum [20] ( Fig. 1b ). Indeed, we can assign σ peaks to electron energy loss spectroscopy (EELS) and Raman-active vibrational modes [21] , [22] , as listed in Table 1 . This implies that the high-field current fluctuations in single HDT molecules are of inelastic origin [23] , [24] , [25] . To verify the possible roles of inelastic excitations of vibration modes of single-molecule junctions on current fluctuations, we conducted σ measurements on Au single-atom chains. Forming 1 G 0 states using the self-breaking method, with a stretching speed of 6 pm s −1 at 4 K, we exhibited 50-point current measurements in a bias range of −0.04 V≤ V b ≤0.04 V. The relatively small bias window was used because Au single-atom contacts tend to become increasingly unstable at bias voltage above 0.05 V presumably because of the local heating and current-induced forces [13] . 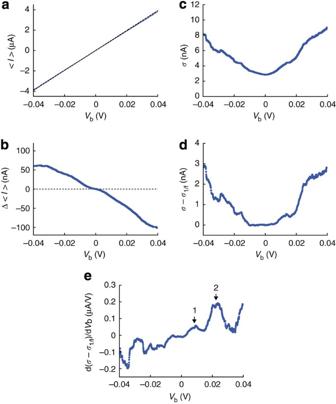Figure 4: Inelastic contributions to electrical conductance and current fluctuations in a single-atom quasi-ballistic chain at 4.2 K. (a) <I>–Vbcharacteristics of an Au single-atom contact at 4 K. The dotted lines are the elastic component. (b) Δ<I> plots derived from the <I>–Vbcurve ina. (c) σ–Vbplots measured for an Au single-atom contact formed at 4.2 K. (d) Plots of (σ–σ1/f) with respect toVband (e) the corresponding noise spectrum. Arrows point to the characteristic peaks in the spectrum at the positiveVbrange measured. < I >– V b plots in Figure 4a show linear characteristics reflecting the quasi-ballistic nature of electron transport through an Au single-atom contact [26] . We extract the inelastic component by examining linear fitting to Figure 4a in a bias range from −0.001 V to 0.001 V. In contrast to HDT molecules demonstrating increased transmission via active inelastic channels, Δ< I >– V b plots in Figure 4b reveal negative contributions of electron–phonon interactions in an Au single-atom chain on the electrical conductance [26] . This discrepancy can be explained by considering the relative importance of the counteracting effects of elastic and inelastic processes in electron transmission through single-atom and molecule junctions; whereas the inelastic mechanism leads to enhanced transmission, elastic contribution involving virtual phonon excitations decreases transmission [27] , [28] , [29] . Theoretical studies have predicted a shift in the balance towards predominance of inelastic effects as transmission T becomes <0.5 and superior elastic effects for T becomes >0.5, the overall tendency of which agrees with the positive and negative Δ< I > acquired for HDT single-molecule junctions with T ~10 −3 and Au single-atom chains with T ~1, respectively [27] , [28] , [29] . As for the high-field current fluctuations, σ shows a stepwise manner analogous to that found for single HDT molecules ( Fig. 4c,d ). The corresponding σ spectrum demonstrates peaks at V p =8 and 22 mV ( Fig. 4e ). Significantly, we again find good accordance between these peak voltages and the characteristic vibration modes of single-atom wires at energies 10 and 18 meV reported in previous scanning tunnelling microscopy studies [30] , [31] ( Table 1 ). It is therefore corroborated that bias voltage-induced conductance fluctuations can serve as a unique molecular signature for single-molecule identifications. Figure 4: Inelastic contributions to electrical conductance and current fluctuations in a single-atom quasi-ballistic chain at 4.2 K. ( a ) < I >– V b characteristics of an Au single-atom contact at 4 K. The dotted lines are the elastic component. ( b ) Δ< I > plots derived from the < I >– V b curve in a . ( c ) σ– V b plots measured for an Au single-atom contact formed at 4.2 K. ( d ) Plots of (σ–σ 1/f ) with respect to V b and ( e ) the corresponding noise spectrum. Arrows point to the characteristic peaks in the spectrum at the positive V b range measured. Full size image The above results strongly indicate that bias voltage-dependent current oscillations are phonon-assisted phenomena relevant to electron vibration interactions in atomic/molecular bridges. Inelastic tunnelling in molecular systems is known to cause a local heating [13] , [32] , [33] , [34] . A certain amount of heat is anticipated to pile up in the molecular junctions every time a new inelastic channel sets in. Although this excess heat dissipates via lattice conduction through two electrodes connecting a molecule, local heating effectively raises the junction temperature T eff above the bath temperature [13] , [32] , [33] , [34] . This may yield a stepwise increase in the thermal noise with increasing V b , which explains a staircase-like increase of σ observed in single HDT molecules and also in Au single-atom wires. It has been theoretically proposed that the heating rate can be deduced by analysing the bias voltage dependence of Johnson–Nyquist noise in molecular junctions [23] , [25] . We therefore sought to extract information regarding electrical heating in HDT junctions from the σ plots in Figure 2d . We evaluated T eff by tentatively considering σ T =(σ–σ 1/f ), where σ T is the thermal noise component of σ, and assuming σ T √ T eff . The relative increase in σ T at V b =0.4 V from the zero-bias value is about 20, from which we obtain T eff ~1,600 K at a bath temperature of 4 K. The estimated T eff is obviously too high and contradicts the fact that an HDT molecule can be held stable during a bias sweep without being burned out. The overestimation of T eff , which is also marked by the fact that the IET spectrum can be observed, suggests significant inelastic noise in the σ–σ 1/f of single HDT molecules derived from the stochastic nature of phonon-assisted electron tunnelling and concomitant fluctuations in the phonon-induced energy levels [24] , [35] , [36] . Shot noise measurements have proven to be a powerful method for evaluating Fano factors, as well as the number and transparency of charge transmission channels in atomic/molecular conductors [9] , [10] , [37] . A theoretical model predicts a linear increase in the power spectral density of this shot noise with the bias voltage in a quasi-ballistic Au single-atom chain under a condition T eff > hν / k B , where ν is the frequency of phonon modes [38] . Indeed, we found a stepwise linear increase in σ–σ 1/f after each vibration mode excitation above 0.01 V, as shown in Figure 2e , which in turn suggests a significant local heating in an Au chain that raises its T eff to > hν / k B ~230 K at V b =0.02 V by virtue of the poor contact-cooling efficiency via lattice heat conduction at 4 K. Furthermore, the positive contributions of inelastic channels to noise amplitude found in the present study suggest a weak electron–phonon interaction and symmetric molecule–metal electronic coupling in HDT single-molecule junctions [35] . (It should be noted that our discussions on inelastic noise is based on a fixed sampling rate. Although the noise amplitude is anticipated to change at different data acquisition speeds, the qualitative arguments on the voltage-specific change in noise amplitudes attributable to the electron–vibration interactions in atomic/molecular conductors still hold.) These results indicate that vibrational mode-specific inelastic noise in single molecules can be more than a useful molecular signature to identify single-molecule junctions: with elaborate theoretical models, it can serve as a unique probe for detailed investigation of the electronic properties of single-molecule bridges. Fabrication of mechanically controllable break junctions (MCBJs) Lithographically defined nano-MCBJs were exploited to form single-molecule bridges. Fabrication procedures of nano-MCBJs are described elsewhere [26] . In short, we spin-coated a polyimide on a phosphor bronze substrate for electrical insulation. Sub-micrometer-scale Au junctions were then patterned using an electron beam lithography technique and subsequent lift-off processes. The sample was then exposed to reactive ion etching to remove polyimide underneath the junctions. As a result, we obtained Au nanobridges with free-standing length of about 2 μm. In experiments, we first bent a substrate with a three-point bending mechanism and ruptured Au junctions immersed in a dilute toluene solution of test molecules. The sample geometries were designed to provide the damping factor r =Δ d /Δ L ~3×10 −4 , where Δ d and Δ L denote the displacements of the MCBJ electrodes and the substrate deflection, respectively [19] . Here, we used HDTs, benchmark molecules the electron transport properties of which have been studied intensively [39] , [40] . Subsequently, we evacuated the sample chamber to remove the solvent, leaving HDT molecules adsorbed on a fresh fracture surface of Au junctions. When the vacuum level reached below 10 −5 torr, we performed opening and closing of Au junctions repeatedly for hundreds of cycles at room temperatures. At the same time, we examined the evolution of Au–HDT–Au structures by monitoring temporal conductance changes of junctions under a junction-stretching speed ν d of 0.6 pm s −1 using a picoammeter (Keithley 6487) under a DC bias voltage of 0.2 V. The measured G - t curves revealed conductance steps at <1 G 0 , suggestive of formations of Au–HDT–Au systems ( Supplementary Fig. S1 ). After this, we slowly cooled the junctions to 4 K. Formations of Au–HDT–Au single-molecule bridges We created an HDT single-molecule bridge using a self-breaking method [9] under ν d =6 pm s −1 and V b =0.2 V at 4 K. Conductance decreased in a stepwise manner. We stopped junction stretching when a well-defined G -plateau at 1.3×10 −3 G 0 was detected right after a conductance drop from 1 G 0 , which indicates opening of an atom-sized electrode gap ( Supplementary Fig. S2 ). Inelastic electron tunnelling spectroscopy measurements To verify the presence of HDT molecules between two electrodes, we exhibited inelastic electron tunnelling spectroscopy (IETS) analyses by measuring d I /d V b in a bias range of 0.4 V≤ V b ≤0.4 V using a lock-in amplifier (SR830, Stanford Research Systems) with a reference AC voltage of 10 m V rms at 1 kHz after forming and holding the single-molecule conductance state ( Supplementary Fig. S3 ). The differential conductance was found to increase in a stepwise manner with V b , indicating the opening of inelastic channels. d 2 I /d V b 2 – V b characteristics were obtained numerically from the measured d I /d V b curves. Pronounced peaks were observed in the IET spectrum that can be assigned to the IETS-active vibrational modes of Au–alkanedithiol–Au bridges. How to cite this article: Tsutsui, M. et al. Single molecule identification via electric current noise. Nat. Commun. 1:138 doi: 10.1038/ncomms1141 (2010).